Aharonov–Bohm effect in the tunnelling of a quantum rotor in a linear Paul trap Quantum tunnelling is a common fundamental quantum mechanical phenomenon that originates from the wave-like characteristics of quantum particles. Although the quantum tunnelling effect was first observed 85 years ago, some questions regarding the dynamics of quantum tunnelling remain unresolved. Here we realize a quantum tunnelling system using two-dimensional ionic structures in a linear Paul trap. We demonstrate that the charged particles in this quantum tunnelling system are coupled to the vector potential of a magnetic field throughout the entire process, even during quantum tunnelling, as indicated by the manifestation of the Aharonov–Bohm effect in this system. The tunnelling rate of the structures periodically depends on the strength of the magnetic field, whose period is the same as the magnetic flux quantum φ 0 through the rotor [(0.99±0.07) × φ 0 ]. The quantum dynamical phenomenon in which a particle tunnels through a barrier that it classically could not penetrate [1] was first investigated in the 1920s to explain alpha decay [2] , [3] . There are also many other natural phenomena ranging from cosmological scales [4] to microscopic scales [5] , such as chemical reactions [6] , that arise from the quantum tunnelling effect; quantum tunnelling effects in artificial materials have been investigated using diodes (tunnel diodes [7] ) and superconductors (Josephson junctions [8] , [9] , [10] , [11] ) and have been achieved in quantum simulators [12] , [13] . Determining the dynamics of quantum tunnelling is a difficult task because the momentum during quantum tunnelling might be purely imaginary [14] , and it is the tunnelling probability that is usually calculated instead [15] , [16] . However, the dynamics of tunnelling particles can be investigated if one can construct a highly coherent tunnelling system. Trapped ions form a highly controllable, isolated quantum system in which both the internal and motional degrees of freedom have long coherence times [17] . Using one-dimensional (1D) ion chains trapped in a linear Paul trap, the oscillation can be cooled to near the ground states, and phonon manipulation can be achieved through laser irradiation [18] . An important feature of a trapped-ion system is the coulomb interaction between ions, which generates an effective interaction between ions for quantum information processing [17] . By virtue of these characteristics, a trapped-ion system is one of the more promising candidates for quantum information processing [17] . However, the coulomb interaction also provides several types of spatial arrangements of the trapped ions, that is, Wigner crystals, including 2D structures [19] . So far, the phase transitions [20] , [21] and dynamics [22] of these Wigner crystals have been investigated both theoretically and experimentally. However, these experiments have not been performed in the quantum regime [22] , [23] because the motions of such 2D structures have never been cooled to near the ground states. The Aharonov–Bohm (AB) effect [24] , in which a charged particle is affected by a magnetic field even as it travels through a region in which the magnetic field is zero, has been experimentally confirmed using an electron in a superconducting ring [25] , [26] and other materials [27] , [28] , [29] , [30] . Even in a non-localized magnetic field, the wave function of a charged particle obtains a phase that is proportional to the area of a closed loop [31] , [32] . This effect is also referred to as the AB effect. Charged quantum tunnelling particles should be affected by the vector potential of a magnetic field even during quantum tunnelling. Thus, the AB effect should occur for tunnelling particles and is an example of the dynamics of tunnelling particles. In this study, we have realised a quantum tunnelling rotor, which consists of three ions and has a 2D structure that is cooled to near the motional ground state in a linear Paul trap. This rotor has two stable orientations and can transition from one to another though quantum tunnelling. Because of the controllability and simplicity of the trapped-ion system, this quantum tunnelling rotor may offer a novel approach to understanding quantum tunnelling dynamics, and we were successful in observing the AB effect of tunnelling particles using this system. Several recent technical advancements regarding the manipulation of ions, such as gate operations and coherent motional controls [17] , [18] , offer further means of controlling the quantum tunnelling rotor. The quantum tunnelling rotor A linear Paul trap, whose normal-mode frequencies are comparable along two axes ( x , z ) and large along the remaining axis ( y ), can be used to trap a single triangular structure of three 40 Ca + ions ( Fig. 1a ) [18] , [19] . The symmetry of the potential defines two stable orientations for the triangular structure, which are referred to here as ‘up’ and ‘down’, and the motional modes of these structures are more complex than those of a 1D coulomb chain [20] . Of the four lowest energy modes represented in Fig. 1b , the mode indicated by the solid curve represents a ‘rotational mode’ in which the ions rotate around the centre of the triangular structure. Here we demonstrate the cooling of the rotational mode, which is one of the 2D modes, to near the ground state. Theoretically, the rotational mode has interesting characteristics: its normal-mode frequencies become zero at critical points, which corresponds to ω x =2 π × 1.119 MHz in Fig. 1b . Under such conditions, the rotational mode becomes massless, and singular phenomena that are similar to other degrees of freedom of 2D structures in a linear Paul trap are expected [21] . 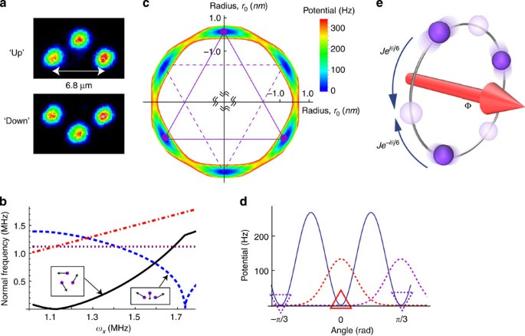Figure 1: The quantum tunnelling rotor. (a) Charge-coupled device images of the two degenerate triangular crystal structures. (b) Calculated energies of the four lowest eigenmodes. The solid curve corresponds to the rotational mode, and the dashed curve corresponds to the zigzag mode. The dot-dashed and dotted curves represent the energies of the centre-of-mass modes of the radial and axial directions, respectively. The left- and right-hand insets display the sets of displacement vectors for the rotational and zigzag modes, respectively. The normal-mode frequency in the axial direction isωz=2π× 1.119 MHz. (c) The quantum tunnelling rotor indicated the potential energy and pattern diagrams of the quantum tunnelling of a three-ion triangular structure. (d) The solid blue curve represents the potential energy as a function of the rotational angle. The red (purple dashed) triangle corresponds to one of the bound states in the well, as denoted by ‘up’ (‘down’) ina, and the dashed red (purple) curve represents the corresponding wave function. (e) A charged quantum rotor in a magnetic field. The sign of the AB phases is dependent on the direction of rotation, whereθ(=6π(Φ/φ0)) is the AB phase for tunnelling. Figure 1: The quantum tunnelling rotor. ( a ) Charge-coupled device images of the two degenerate triangular crystal structures. ( b ) Calculated energies of the four lowest eigenmodes. The solid curve corresponds to the rotational mode, and the dashed curve corresponds to the zigzag mode. The dot-dashed and dotted curves represent the energies of the centre-of-mass modes of the radial and axial directions, respectively. The left- and right-hand insets display the sets of displacement vectors for the rotational and zigzag modes, respectively. The normal-mode frequency in the axial direction is ω z =2 π × 1.119 MHz. ( c ) The quantum tunnelling rotor indicated the potential energy and pattern diagrams of the quantum tunnelling of a three-ion triangular structure. ( d ) The solid blue curve represents the potential energy as a function of the rotational angle. The red (purple dashed) triangle corresponds to one of the bound states in the well, as denoted by ‘up’ (‘down’) in a , and the dashed red (purple) curve represents the corresponding wave function. ( e ) A charged quantum rotor in a magnetic field. The sign of the AB phases is dependent on the direction of rotation, where θ (=6 π (Φ/ φ 0 )) is the AB phase for tunnelling. Full size image Near the critical point of the rotational mode ( Fig. 1b ), the wave functions of each ion in the rotational direction are elongated, and quantum tunnelling can occur between two degenerate triangular structures [33] . Because the other motional modes have much larger spring constants by virtue of the strong coulomb interaction, it is reasonable to assume that these modes are unaffected by the quantum tunnelling. These triangular structures become a quantum rigid rotor, which is a quantum system that has a rotational degree of freedom but maintains its structure. In this system, the rotation of the quantum rigid rotor is driven by the quantum tunnelling. We refer to this system as a ‘quantum tunnelling rotor’ ( Fig. 1 ). Ions also have internal degrees of freedom, that is, spins, and the tunnelling can depend on the spin states of the ions of the quantum tunnelling rotor [33] . Using this system, we can investigate and manipulate the tunnelling system itself by controlling the trap parameters and the spin state. Figure 1c,d illustrates the effective potential of the quantum tunnelling rotor in the linear Paul trap for the actual experimental parameters used. Each bound state in the periodical multi-well potential corresponds to a single stable orientation of the quantum tunnelling rotor. In addition, the overlap of the up and down wave functions of the ions observed in Fig. 1d indicates that quantum tunnelling is possible. The orientations of the atomic triangles in this condition are not stable under laser-cooled temperatures. However, under intermediate radial confinement conditions, corresponding a normal frequency of ω x =2 π × 1.523 MHz in Fig. 1b , both degenerate triangular structures are stable even for ‘hot’ Doppler-cooled temperatures. Thus, projective measurements of the triangle orientations can be performed. Observation of quantum tunnelling We experimentally observed the quantum tunnelling of the rotor using a magnetic field of a certain magnitude. The three ions were trapped in a linear Paul trap with normal-mode frequencies of { ω x , ω y , ω z }=2 π × {1.523, 1.961, 1.119} MHz (further details of the experimental system can be found in refs 34 , 35 ), and the orientation of the triangular structure could be set using intermediate confinement conditions. 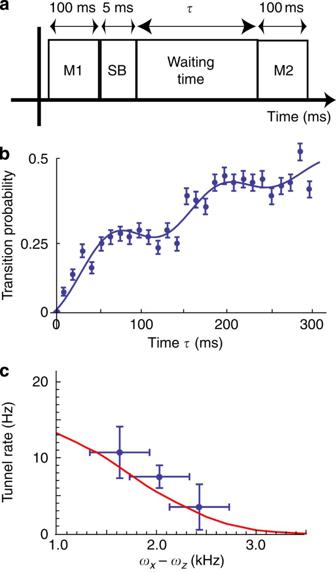Figure 2: Quantum tunnelling in the rotor. (a) Experimental time sequences. M1: measurement of the initial state, SB: sideband cooling of the rotational mode and M2: measurement of the final state. (b) The correlation between the initial and final states from 400 experiments per data point as a function of the waiting timeτ. The fit function is the sum of a sinusoidal curve and an exponential decay. The error bars represent the s.d. of binomial distributions. (c) The tunnelling rate as a function of the radial confinement. The solid curve represents a numerical calculation performed using the experimental parameterωz=2π× 1.119 MHz. The vertical error bars represent the s.e. of fitting. The horizontal error bars correspond to the s.d. of the amplitude of the trap RF. Figure 2a shows the time sequence of the experiment, which began with the measurement of the initial state of the triangular structure using a charge-coupled device camera. For quantum tunnelling to be observed, it was necessary to cool the quantum tunnelling rotor to the rotational ground state. The rotational mode had the lowest heating rate among the 2D motional modes (see Methods section) and could be cooled to near the motional ground state (a mean phonon number of n rt =0.088±0.007) using the sideband cooling technique. After cooling, the trap radio frequency (RF) was adiabatically reduced to create the quantum tunnelling rotor. At that time, the normal-mode frequency of the rotational mode changed to 2 π × 0.18 kHz from 2 π × 750 kHz ( Fig. 1b ). There was a small amount of heating of the quantum tunnelling rotor caused by noise, micromotion and diabaticity when the trap potential was changed. Under tunnelling conditions, we assumed the mean phonon number to be n rt ~\n4 (see Methods section). After a time τ , the trap RF was increased, and we again measured the orientation of the triangular structures. Near the critical point, the quantum tunnelling rotor in the rotational ground state oscillated between the two degenerate orientations because of the quantum tunnelling ( Fig. 2b ). Figure 2: Quantum tunnelling in the rotor. ( a ) Experimental time sequences. M1: measurement of the initial state, SB: sideband cooling of the rotational mode and M2: measurement of the final state. ( b ) The correlation between the initial and final states from 400 experiments per data point as a function of the waiting time τ . The fit function is the sum of a sinusoidal curve and an exponential decay. The error bars represent the s.d. of binomial distributions. ( c ) The tunnelling rate as a function of the radial confinement. The solid curve represents a numerical calculation performed using the experimental parameter ω z =2 π × 1.119 MHz. The vertical error bars represent the s.e. of fitting. The horizontal error bars correspond to the s.d. of the amplitude of the trap RF. Full size image Magnetic field dependency of quantum tunnelling The AB effect must occur in the quantum tunnelling rotor in a magnetic field because the dynamics of the quantum tunnelling rotor are governed by the quantum interference of two-directional rotations; see Methods section for details. Thus, the tunnelling of the quantum tunnelling rotor can be controlled by adjusting the strength of the magnetic field. The dependency of the transition probability on the number of magnetic flux quanta was investigated by fixing the waiting time to 50 ms and adiabatically varying the magnetic field, with the field held constant during tunnelling ( Fig. 3 ). The detail of the experimental setup regarding the magnetic fields are presented in Methods section. The oscillation period estimated from a sinusoidal fit is (0.99±0.07) φ 0 , for the single magnetic flux quantum φ 0 = h / e , where h is the Planck constant and e is the elementary charge. This fitting result agrees with the theoretically predicted oscillation period obtained from equation (6), which is presented in the Methods section. 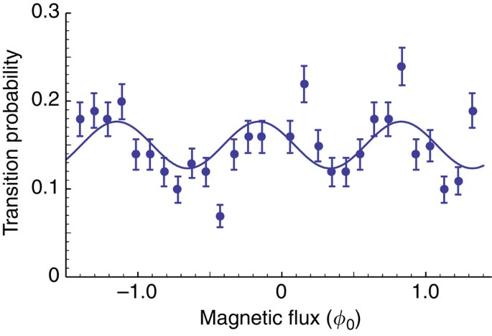Figure 3: The Aharonov–Bohm effect during quantum tunnelling. The transition probability as a function of the magnetic flux produced by the tunable coils expressed in magnetic quantum units (φ0=4.14 × 10−15Wb). We performed 800 experiments per data point. The error bars are statistical errors calculated by assuming binomial distributions of the results. The solid curve represents a cosine fit to the results. Figure 3: The Aharonov–Bohm effect during quantum tunnelling. The transition probability as a function of the magnetic flux produced by the tunable coils expressed in magnetic quantum units ( φ 0 =4.14 × 10 −15 Wb). We performed 800 experiments per data point. The error bars are statistical errors calculated by assuming binomial distributions of the results. The solid curve represents a cosine fit to the results. Full size image Figure 2b presents the experimental results for the tunnelling dynamics of the rotor. These dynamics can be divided into quantum tunnelling and classical rotation. The ions are not completely in the ground state; ions in the rotational excited states rotate without tunnelling because the energies of these states are greater than the potential barrier, whose height is h × 250 Hz ( Fig. 1d ) where h is the Planck constant. The transition probabilities of the tunnelling consist of two components. One component represents the tunnelling between the up and down states and can be described by a sinusoidal curve, and the other represents the rotation of the excited states and can be described by an exponential decay. A fit of the experimental data to a sum of these two curves yields a tunnelling rate of 7.6±0.3 Hz and a decay time constant of 5.4±0.3 s −1 , for example, the mean rates of the classical rotation. The amplitude of the oscillation, which was determined to be 0.19 based on the thermal distribution of the phonon number, is consistent with the population of the ground state. Furthermore, our tunnelling rates for different radial confinements ( Fig. 2c ) exhibit good agreement with the numerical solution of the Schrödinger equation for the potential illustrated in Fig. 1d . The oscillation in the transition probability can therefore be attributed to quantum tunnelling. Figure 3 shows the strength of the magnetic field dependency of the tunnelling rate. This figure demonstrates that the ions couple to the vector potential even under quantum tunnelling conditions; that is, the system exhibits the AB effect. The amplitude of the oscillation is also consistent with the quantum tunnelling result ( Fig. 2b ). Note that the AB effect does not occur in classical rotations of the excited states because of the incoherency. The quantum tunnelling rotor may be affected by the Lorentz force during quantum tunnelling. The Lorentz force can be calculated from a velocity and a magnetic field. The expectation value of the particle position can be evaluated using Ehrenfest’s theorem; however, the velocity of a tunnelling particle is expected to be purely imaginary because E − U is negative (where E is the kinetic energy and U is the potential energy). One approach to circumventing this difficulty is to take the absolute value | E − U | to be the tunnelling kinetic energy. The validity of this approach is supported by quantum clock conditions [15] , the Ehrenfest theorem [36] and an analogous experimental demonstration using a single photon [14] . Using this approach, we estimate the effective maximal rotation speed v of the rotor to be (2| U 0 − E |/ M ) 1/2 (refs 14 , 15 , 36 ). Here, U 0 = h × 270 Hz is the maximal potential energy ( Fig. 1d ), E = h × 90 Hz is the energy of the rotational ground state and M =3·40·1.67 × 10 −27 kg is the mass of the quantum tunnelling rotor. This speed yields a maximal strength of the Lorentz force of evB ~\n10 −26 N for a magnetic field of B ~\n5 G. An alternative approach is to calculate the effective mean velocity v m from the tunnelling rate. In this case, v m = Jr 0 π /3, where J =7.4 Hz is the tunnelling rate and r 0 =3.42 mm is the radius of rotation. This velocity yields a mean strength of the Lorentz force of ev m B ~\n10 −27 N for the same magnetic field. According to the results of both approaches, the Lorentz force is quite small and can be ignored in our experiment because the Lorentz-force-induced change in the radius of the closed loop would be on the order of femtometres. Quantum tunnelling rotor in a magnetic field The AB effect occurs in the quantum tunnelling rotor, and the wave functions of the ions gain a phase that is proportional to the homogeneous magnetic field and the area of the closed loop drawn by the path of each ion of the quantum tunnelling rotor [31] , [37] . Because of the strong radial confinement of each ion, this closed loop corresponds to the potential valley shown in Fig. 1c . The wave function of the quantum tunnelling rotor can be expressed as [38] where ψ up, down ( t ) are the wave functions of the two quantum tunnelling rotor orientations, Δ t is a short time interval and J r ( J l ) is the complex amplitude of the tunnelling for clockwise (anti-clockwise) rotation. Because the AB effect introduces a phase difference between the clockwise and anti-clockwise rotations ( Fig. 1e ) and the quantum tunnelling rotor has sixfold rotational symmetry, the complex amplitudes are given by where J is the strength of the tunnelling, Φ= SB ⊥ is the magnetic flux that penetrates the quantum tunnelling rotor, S is the area of the closed loop, B ⊥ is the magnetic field component perpendicular to the plane of the quantum tunnelling rotor, φ 0 = h / e is a quantum of magnetic flux, h is the Planck constant and e is the elementary charge. Using these amplitudes, the wave function of the up orientation is given by where the transition probability P from ψ up to ψ down (and vice versa) is calculated as using Fermi’s golden rule. The tunnelling dynamics depends on the magnetic flux with a period given by φ 0 . Detection Images were acquired from the direction by directing the incident Doppler cooling laser along the direction. The setup and trapped structures are depicted in Fig. 4 . A 1D coulomb chain was observed for strong confinement conditions (a normal-mode frequency of ω x >2 π × 1.75 MHz in Fig. 1b ), whereas near intermediate confinement ( Fig. 4c,d ), the orientation of the triangular structure did not change during Doppler cooling. The orientations of the triangles in these two cases could be distinguished within a detection time of 50 ms. 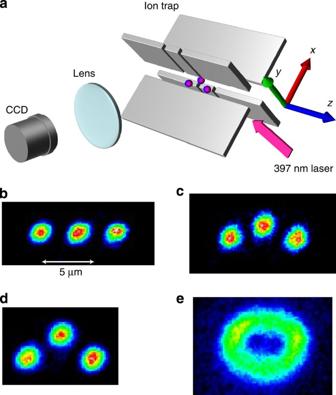Figure 4: Experimental system. (a) The relative geometry of the ion trap and the imaging system. Images were acquired of three40Ca+ions under various conditions: (b) under strong confinement conditions (ωx=2π× 2.1 MHz), (c) under slightly stronger than intermediate confinement (ωx=2π× 1.65 MHz), (d) under intermediate confinement conditions (ωx=2π× 1.523 MHz) and (e) near the critical point (ωx=2π× 1.119 MHz). Figure 4: Experimental system. ( a ) The relative geometry of the ion trap and the imaging system. Images were acquired of three 40 Ca + ions under various conditions: ( b ) under strong confinement conditions ( ω x =2 π × 2.1 MHz), ( c ) under slightly stronger than intermediate confinement ( ω x =2 π × 1.65 MHz), ( d ) under intermediate confinement conditions ( ω x =2 π × 1.523 MHz) and ( e ) near the critical point ( ω x =2 π × 1.119 MHz). Full size image Even under intermediate confinement conditions, the triangular orientation was not stable against background-gas collisions (300 K). However, because of the ultra-high vacuum, the collision rate of such collisions is ~\n1 every few minutes and was thus sufficiently slow that the orientations could be detected. Stabilization of the trap RF Because the tunnelling frequency depends on the normal-mode frequencies, the trap RF and radial potential must be stabilised. The amplitude of the trap RF was monitored using a pick-up coil and an RF power metre, and the trap RF was stabilised using a feedback technique. The fluctuations of the normal-mode frequencies were less than a few hundred hertz. Sideband cooling The sideband cooling of 2D structures in a linear Paul trap is difficult to achieve because the ions are subject to large micromotions when they are not located at the node of the trap RF. However, we were able to cool the rotational mode to near the ground state using sideband cooling with a red sideband transition laser ( 2 S 1/2 − 2 D 5/2 ; 729 nm) and a quenching laser ( 2 D 5/2 − 2 P 3/2 ; 854 nm). The lasers were simultaneously incident on the trap for 5 ms. The asymmetry between the red and blue sideband spectra after sideband cooling ( Fig. 5 ) indicated cooling to near the ground state. 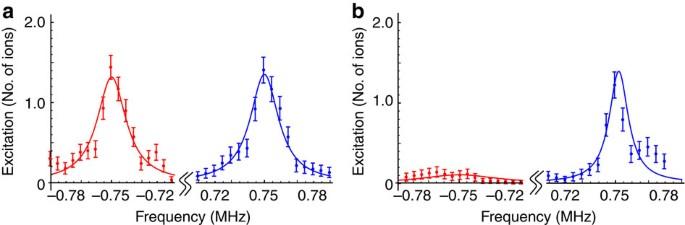Figure 5: Sideband spectra of the rotational mode. Rotational blue and red sideband spectra (a) before and (b) after sideband cooling. The number of excitations of the three ions is presented as a function of the frequency. We performed 200 experiments per data point. The error bars represent the s.d. of binomial distributions. Figure 5: Sideband spectra of the rotational mode. Rotational blue and red sideband spectra ( a ) before and ( b ) after sideband cooling. The number of excitations of the three ions is presented as a function of the frequency. We performed 200 experiments per data point. The error bars represent the s.d. of binomial distributions. Full size image Adiabatic cooling The ground state of the rotational mode must be prepared to observe quantum tunnelling, and because the normal-mode frequency of the rotational mode is quite small under tunnelling conditions, an extremely low temperature is necessary to achieve this goal. To obtain a ground-state population larger than 0.1, a temperature of <90 nK is required; this temperature is much lower than the recoil limit in conventional sideband cooling. Adiabatic cooling, which has been demonstrated with trapped ions [39] , was therefore performed to achieve the ground state. Reducing the energy of a single motional quantum ℏ ω under adiabatic conditions reduces the temperature, even though the phonon entropy is conserved. The mean phonon number at temperature T is calculated using boson statistics as follows: where ω is the secular frequency of the mode, k B is the Boltzmann constant and ℏ is the reduced Planck constant. In the experiment, the mean phonon number of the rotational mode just after sideband cooling was 0.08, which corresponds to 10 mK. We reduced the secular frequency adiabatically from 750 to 0.18 kHz to reduce the temperature to 40 nK, although there was some heating, as indicated by an increase in the entropy of the motional mode. This temperature was sufficiently cold for quantum tunnelling to be observed. Heating Heating of the trapped ions causes a decrease in the population of the ground state of the quantum tunnelling rotor. For the intermediate confinement state, we observed a heating rate after sideband cooling that was much less than 1 quantum s −1 , and no heating of the rotational mode was observed within 1 s under these conditions. Determining the mean phonon number after a time interval of 1 s was difficult because the other modes were subject to stronger heating. This lack of sensitivity can be attributed to the symmetry of the rotational mode. It is difficult for electric field noise to heat the rotational mode because the electrodes are separated from the rotor by distances that are much larger than the rotor’s own length scale. The other modes, for example, the zigzag mode, could not be cooled by the sideband cooling because of its strong heating. We measured the phonon number of the rotational mode after ramping down the potential to create the triangular structure of the quantum tunnelling rotor and then ramping it back up to its original magnitude. After the potential was ramped up, the mean phonon number was 8. This value was nearly independent of the waiting time between ramping down and up for times of up to 300 ms. Hence, we speculate that the heating of the rotational mode predominantly occurred during the variation of the potential. Although the trap frequencies were very low near the critical points, the heating rate for the rotational mode remained small. This low heating was also likely attributable to the symmetry of the rotational mode. However, this value depended on the position of the centre of the triangular structure. The origins of the heating of the rotational mode may have been trap RF, other hot modes and various sources of noise. These heating sources were carefully eliminated by changing the position of the rotor. Thus, it is possible that fine control of the DC voltages of the linear Paul trap in synchronisation with the variation of the amplitude of the trap RF may permit the preparation of a quantum tunnelling rotor that is colder than that of the current experiment. Magnetic field To ensure that the magnetic field was sufficiently stable for sideband cooling, we used two orthogonal sets of coils to generate the magnetic fields. The first set created a constant magnetic field (3.4 G) for the sideband cooling and an offset of the magnetic flux, whose directional vector was . Here, the normal vector of the triangular structure was taken to be {0, 1, 0} (see Fig. 4a ). The second set of coils created a tunable magnetic field whose direction was to change the number of magnetic flux quanta penetrating the quantum tunnelling rotor. From the area of the closed loop (37 μm 2 ) and the direction of the magnetic field, the number of magnetic flux quanta that penetrated the quantum rotor was Φ/ φ 0 =1.5±0.2 when there was no current flowing through the tunable coils. This value is subject to certain errors because of the unknown residual magnetic fields and the angular error between the coils and the triangular structure of the ions. Fitting The fit to the transition-probability data presented in Fig. 2b is given by where p 0 is the population of the rotational ground state of the quantum tunnelling rotor, ν is the tunnelling frequency, T 2 is the coherence time of the tunnelling and ε is the average rotational velocity of the rotational excited states. Fitting parameters of p 0 =0.10±0.02, ν =7.6±0.3 Hz, T 2 =300±200 ms and ε =5.4±0.3 s −1 were used. The coherence time may have been limited by the heating of the rotational mode and by fluctuations in the tunnelling rate. According to Fig. 2c in the main text, the tunnelling rate ν was near the experimental condition ω x − ω z ~\n2 π × 2 kHz. If the fluctuation in the radial confinement is assumed to have been ~\n300 Hz because of imperfections in the feedback control of the trap RF, the fluctuations in the tunnelling frequency were 2.4 Hz. This indicates that if we consider only tunnelling rate fluctuations, the coherence time was 130, which is consistent with the fitting parameter. The fit function used to obtain the results presented in Fig. 3 in the main text was where n is the number of magnetic flux quanta penetrating the quantum tunnelling rotor. The fitting parameters were a =0.06±0.02, ξ =0.99±0.07, θ 0 =0.28 π ±0.22 π and h =0.15±0.01. How to cite this article: Noguchi, A. et al . Aharonov–Bohm effect in the tunnelling of a quantum rotor in a linear Paul trap. Nat. Commun. 5:3868 doi: 10.1038/ncomms4868 (2014).